Unique distal size selectivity with a digold catalyst during alkyne homocoupling Metal-catalysed chemical reactions are often controlled by steric hindrance around the metal atom and it is rare that substituents far away of the reaction site could be differentiated during reaction, particularly if they are simple alkyl groups. Here we show that a gold catalyst is able to discriminate between linear carbon alkynes with 10 or 12 atoms in the chain during the oxidative homocoupling of alkynes: the former is fully reactive and the latter is practically unreactive. We present experimental evidences, which support that the distal size selectivity occurs by the impossibility of transmetallating two long alkyl chains in an A-framed, mixed-valence digold (I, III) acetylide complex. We also show that the reductive elimination of two alkyne molecules from a single Au(III) atom occurs extremely fast, in <1 min at −78 °C (turnover frequency>0.016 s −1 ). Organic synthesis takes advantage of the predictable outcome of reactions where bulky groups are involved. Metal-catalysed carbon–carbon bond-forming reactions are not an exception since they are generally controlled by the steric hindrance around the catalytic site, which is given by the bulkiness of the ligands or the reactants, rather than for substituents far away from the reactive site. It is rare that substituents at more than six atoms distance from the reactive site can be sterically differentiated during catalysis [1] , [2] . Here we show a gold catalyst that is able to discriminate between linear chain alkynes only differing in one ethylene group at an eight-carbon distance of the catalytic site. This level of discrimination is extraordinary and difficult to achieve even for rigid microporous solid frameworks [3] , [4] , [5] . Gold catalysis has been intensively studied during the last decade and, in particular, the use of the redox pair Au(I)/Au(III) has arisen much interest among chemists as a catalyst for new carbon–carbon and carbon–heteroatom bond-forming reactions [6] , [7] , [8] , [9] , [10] . Despite the increasing number of new transformations reported, particularly with alkynes [11] , [12] , fundamental studies covering the elemental steps of the gold-catalysed redox cycle remain scarce [13] , [14] . Here we dissect the fundamental steps during the oxidative coupling of alkynes catalysed by Au(I)/Au(III) to find a reasonable explanation to the distal size selectivity observed. Distal size selectivity of alkynes with gold catalysts Fig. 1 shows the results for the homocoupling of 1-decyne 1a and 1-dodecyne 1b under gold-catalysed conditions. We found that 1-decyne 1a (C 10 ) reacts smoothly under the gold-catalysed conditions, while 1-dodecyne 1b is nearly unreactive for homocoupling (<5% yield after 24 h). Kinetic measurements by gas chromatography–mass spectrometry (GC–MS, see Supplementary Fig. 1 ) show that the initial rate of 1-decyne 1a is 3.5 times higher than 1-dodecyne 1b, and that while 1a smoothly converts over the time to the homocoupling product 2a 1-dodecyne 1b rapidly stops converting to the homocoupled product 2b . Notice that a minor non-catalysed polymerization of the alkyne occurs together with the homocoupling reaction. 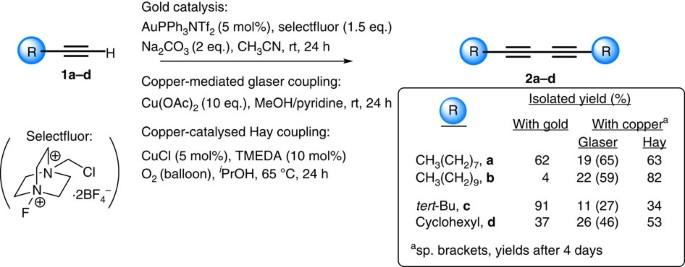Figure 1: Gold or copper-catalysed oxidative homocoupling of terminal alkynes. Notice the different reactivity of alkynes1a–dunder the gold-catalysed conditions reported here and typical copper-catalysed conditions (Glaser or Hay conditions). Isolated yields are the average of two runs. Figure 1: Gold or copper-catalysed oxidative homocoupling of terminal alkynes. Notice the different reactivity of alkynes 1a–d under the gold-catalysed conditions reported here and typical copper-catalysed conditions (Glaser or Hay conditions). Isolated yields are the average of two runs. Full size image Other linear terminal alkynes shorter than 1-decyne 1a (C 6 –C 9 ) react at a similar rate than 1a under gold-catalysed conditions, with final product yields between 60–70%, while 1-undecyne (C 11 ) gives a low yield of homocoupling product (19%) and a longer linear terminal alkyne (C 14 ) is unreactive towards homocoupling. The use of freshly-prepared or just-open commercial bottles of Au catalyst and selectfluor assures reproducible results, otherwise lower yields can be obtained although with still a similar distal size selectivity. This change based on the chain size is remarkable, when moving from 1-decyne 1a (65–80%), then to 1-undecyne (19%) and finally to 1-dodecyne 1b and longer linear alkynes (<5%). It must be highlighted that this distal size selectivity seems to be quite unique with gold, since when the homocoupling of alkynes was carried out under typical copper-mediated (Glaser coupling, that is, the most used protocol for the homocoupling of alkynes in organic synthesis) [15] , [16] or copper-catalysed (Glaser–Hay coupling, with O 2 as the final oxidant) conditions the reaction rate and final yields of 1-decyne 2a and 1-dodecyne 2b are very similar for both alkynes (see Fig. 1 ). These results suggest a profound difference in the mechanism of homocoupling of linear alkynes with gold or copper catalysts. The nearly atomically precise selection of long linear alkynes by gold during the oxidative homocoupling of alkynes is perhaps more striking when we consider alkynes containing bulky substituents at the contiguous positions of the triple bond. For instance, tert- butylacetylene 1c reacts smoothly (91% yield of 2c ) while cyclohexylacetylene 1d gives only a moderate yield of homocoupling product 2d (37% yield). These results clearly contrast with those obtained for copper: while tert -butylacetylene 1c is poorly reactive in the Glaser and Hay couplings (11 and 34% yield after 24 h), cyclohexylacetylene 1d shows a higher reactivity (46% yield after 4 days for the Glaser coupling and 53% yield after 24 h for the Hay coupling) closer to that of long linear alkynes 1a–b . Overall, the results in Fig. 1 clearly show that the gold-catalysed oxidative homocoupling of alkynes occurs with size selectivity along the whole substrate rather than with the classical size selectivity around the reactive site of the substrate, the latter operating in the copper-catalysed reactions. Study of the origin of the distal size selectivity with gold catalysts The elemental steps of the homocoupling of alkynes on gold catalysts (supposing a mixed-valence gold complex) are shown in Fig. 2 and include oxidation of gold(I) to gold (III), formation of the digold complex (approach), transmetallation of the alkyne and reductive elimination [17] , [18] . 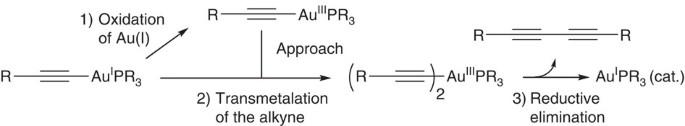Figure 2: Proposed reaction steps for the homocoupling of alkynes on gold catalysts. The reaction pathway includes oxidation of gold(I) to gold (III), formation of the digold complex (approach), transmetallation of the alkyne and reductive elimination17. Figure 2: Proposed reaction steps for the homocoupling of alkynes on gold catalysts. The reaction pathway includes oxidation of gold(I) to gold (III), formation of the digold complex (approach), transmetallation of the alkyne and reductive elimination [17] . Full size image To determine if the first step, that is, the oxidation by selectfluor of the in situ formed gold(I)-acetylide [17] , is responsible for the distal size selectivity observed, the gold(I) acetylides of 1-decyne 1a ( 3a ) and 1-dodecyne 1b ( 3b ) were prepared and a stoichiometric amount of oxidant was added to each of them under the reaction conditions given in Fig. 3 . 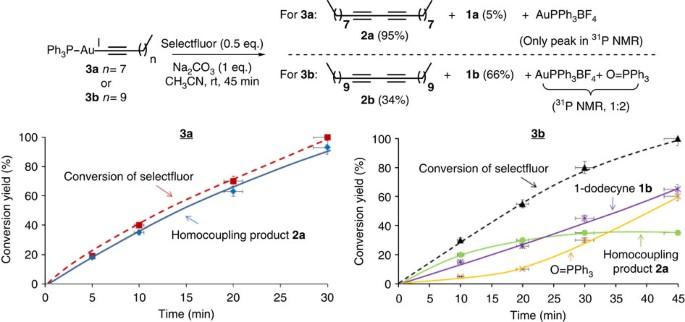Figure 3: Oxidation of gold(I) acetylides by selectfluor. Conversion and yields are calculated on the basis of1H and19F NMR spectroscopy for selectfluor,1H NMR spectroscopy and GC–MS (after extraction of the reaction mixture withn-hexane and addition of dodecane as an external standard) for alkynes and31P NMR spectroscopy for phosphines. Error bars represent an uncertainty of 5% in the value. Figure 3: Oxidation of gold(I) acetylides by selectfluor. Conversion and yields are calculated on the basis of 1 H and 19 F NMR spectroscopy for selectfluor, 1 H NMR spectroscopy and GC–MS (after extraction of the reaction mixture with n -hexane and addition of dodecane as an external standard) for alkynes and 31 P NMR spectroscopy for phosphines. Error bars represent an uncertainty of 5% in the value. Full size image The results show that selectfluor is consumed within 45 min with an initial rate of 250 h −1 for acetylide 3a and 220 h −1 for 3b (measured from the initial slope of the curve and within the timing limitations of the 1 H NMR technique). The reaction rate is expressed in h −1 and increases with the concentration of selectfluor ( Supplementary Fig. 2 ) [17] . While the consumption of selectfluor is similar for the two acetylides 3a–b , the appearance of the homocoupling product is not. For 3a (C 10 ), a new triplet at ~2.1 p.p.m. corresponding to the homocoupling product 2a appears in the 1 H NMR spectra, and this peak increases as selectfluor converts. In contrast, 3b (C 12 ) gives two new signals in the 1 H NMR spectra at ~2.3–2.1 p.p.m., and those signals correspond to the homocoupling product 2b and 1-dodecyne 1b . Extraction of the reaction mixture with n -hexane and analysis by GC–MS and also by 1 H and 13 C NMR spectroscopy confirms that the homocoupling product 2a is the only alkyne product after oxidation of the acetylide of 3a , and that the homocoupling product 2b and free 1-dodecyne 1b in a 1:2 molar ratio are the alkyne products from the acetylide of 3b . The appearance of free alkyne 1b from 3b prompted us to check carefully the spectra of 3a during oxidation, and small amounts (<5%) of free 1-decyne 1a were detected in solution by GC–MS. These results show that the free alkynes 1a or 1b are somehow formed during the oxidation of the Au(I) acetylide complexes 3a–b , respectively. To check if the free alkyne is able or not to enter back the catalytic cycle, an equimolecular amount of 1-dodecyne 1b was added to the C 10 acetylide 3a and then we proceed to oxidize with selectfluor. The results ( Supplementary Fig. 3 ) show that the heterocoupling product C 10 –C 12 4a was formed together with the homocoupling product C 10 –C 10 2a . Complementary 1-decyne 1a was added during the oxidation of the C 12 acetylide 3b , and we found again that the heterocoupling product C 10 –C 12 4a was formed together with the corresponding homocoupling product C 12 –C 12 2b . These results confirm the scrambling of alkynes during reaction. Notice that the homocoupling product of the free alkyne added externally is not obtained in any case, which is in accordance with blank experiments that show that alkyne scrambling between the gold(I) acetylide and a second free alkyne does not occur without any oxidant in the reaction medium. When the two gold(I) acetylides 3a and 3b are combined in a single flask and selectfluor is added, the heterocoupling product 4a is formed in 37% yield, the C 10 –C 10 homocoupling product 2a is formed in 58% yield, the C 12 –C 12 2b is formed in only 5% yield and the free alkyne 1b (50%) persists in solution. These results support that free alkyne is released after oxidation by selectfluor of the acetylide Au(I) complex, that the amount of free alkyne remaining in solution during the coupling is much higher for the C 12 than for the C 10 gold(I) acetylide, and that the released alkyne re-enters into the catalytic cycle. If anhydrous acetonitrile with a 0.5% (v:v) of D 2 O is used as a reaction solvent (instead of non-dried acetonitrile) for the oxidation of 3b , much of the alkyne released (~80%) is d 1 -1-dodecyne 1b– d 1 , which suggests that the released alkyne takes the proton from the solvent. 31 P NMR spectroscopy also shows significant differences during the oxidation by selectfluor of 3a and 3b . For the former (C 10 ), the original peak of phosphine 3a at ~42 p.p.m. disappears as the oxidation converts and the generation of a single new peak at ~32 p.p.m. corresponding to PPh 3 AuBF 4 is observed. In contrast, 3b (C 10 ) shows that the original peak (~42 p.p.m.) is transformed into PPh 3 AuBF 4 (32 p.p.m.) and also into free O=PPh 3 (28 p.p.m.) in a 1:2 molar ratio. Despite homocoupling of the alkyne being incomplete, 1 H and 19 F spectroscopy clearly show the total consumption of selectfluor. Kinetic measurements (see Fig. 3 above) show that as soon as the formation of the homocoupling C 12 product 2b stops during the oxidation of 3b with selectfluor, the formation of free O=PPh 3 increases. A new downshifted peak attributable to a phosphine oxide-gold complex was found during reaction by 31 P NMR spectroscopy ( Supplementary Fig. 3 ). No additional 31 P peaks were found during oxidation, which suggests that phosphine ligands are not detached during reaction, at least at a measurable rate, and that transmetallation (if occurs) and reductive elimination are much faster processes than gold(I) oxidation since no phosphine intermediates are detected. These results indicate that the oxidation of the phosphine follows the oxidation of gold(I) to gold(III), and when the former occurs the active acetylide gold species decompose to O=PPh 3 , free terminal alkyne and gold [19] , [20] . In any case, the results showed above are consistent with the oxidation by selectfluor of the gold(I) acetylide complex independently of the size of the alkyne, with release of homocoupling product and also of free alkyne into the solution. This free alkyne is able to re-enter into the catalytic cycle provided the gold active species is still active. In the case of the C 10 acetylide 3a , the amount of free alkyne 1a detected in the solution is very low and the main alkyne product is the homocoupling product 2a . In contrast, the C 12 acetylide 3b leaves significant amounts of 1-docecyne 1b in solution which, at the end, does not form back productive acetylide gold complex for further homocoupling, at least at a rate that could compete with the destruction of the gold catalyst by oxidation of the metal ligand PPh 3 to O=PPh 3 . The results in Figs 1 and 3 suggest that the distal size selectivity observed for gold occurs after oxidation, when both species Au(I) and Au(III) are already present in the reaction medium. Previous mechanistic studies unveiled that the gold-catalysed oxidative homocoupling of alkynes in solution proceeds through a bimetallic Au(I)/Au(III) acetylide transition state [17] , and density functional theory calculations confirm the feasibility of a digold intermediate species ( Supplementary Fig. 4 ). The digold intermediate sets the Au(I)/Au(III) cations in position and, as a consequence, the alkynes are oriented in a cisoid conformation. If one compares this reaction intermediate for gold with that widely accepted for copper [21] consisting in a tetrahedrically coordinated dimeric Cu(II) acetylide species with the alkynes oriented in opposite directions, one can attempt to explain the different behaviour of gold and copper on the basis of the different geometries. To assess if the spatial approaching of the two gold atoms has any influence on the reaction outcome, three different diphenylphosphine-bridged digold(I) complexes 5a–c with one (methylene), two (ethylene) and three (propylene) methylene units in the tether were prepared ( Supplementary Fig. 5 and Supplementary Discussion ) [22] , [23] . X-ray Diffraction together with cyclic voltammetry studies showed that while 5a presents aurophilic bonding between two gold atoms [14] , 5c has no aurophilic bonds at all [14] and 5b has an intermediate behaviour, depending on the counteranion [24] , [25] . The results indicate that aurophilic bonding has a positive influence on the reaction rate but none on the distal size selectivity. Since previous kinetic studies have demonstrated that the rate-determining step of the gold-catalysed homocoupling of alkynes in solution is the oxidation of gold(I) [17] , it is not surprising that aurophilic bonding improves the reaction rate by neighbouring gold atom-assisted oxidation of gold(I) [26] , [27] . To test if aurophilic bonding has also any influence in the distal size selectivity, we prepared the digold acetylide complexes 6a [Au 2 dppe(C 10 ) 2 ] and 6b [Au 2 dppe(C 12 ) 2 ], and the results after oxidation with selectfluor were compared with those obtained before for the corresponding monogold acetylides 3a–b . The results were nearly identical, with the same amounts of homocoupling products 2a (>95%) or 2b (45%) obtained, and free alkyne 1-dodecyne 1b (~50%) released into solution for the case of the dodecynyl acetylide 6b . Cyclic voltammetry ( Supplementary Figs 6 and 7 and Supplementary Discussion ) confirmed that, in all the complexes tested, oxidation of Au(I) to Au(III) occurs without detecting any Au(II) species [9] , [16] , [23] , [28] . These results validate the mixed-valence digold intermediate Int–1 and clearly show that aurophilic bonding improves the reaction rate but that it is not involved in the distal size selectivity. The reductive elimination from Au(III) complexes to form new C sp 3 − X and C C sp 2 − X bonds (X=heteroatom, C sp 2, C sp 2 , . . . ) is a well-known process [13] , [29] , [30] , [31] , [32] that has been recently reported to occur very rapidly (even at −52 °C) [33] , faster than in palladium (II). Au(III) intermediates have been isolated and characterized [34] , [35] , [36] . Despite the great body of work reported in the literature for alkynes and gold, the reductive elimination of C sp bonds from Au(III) complexes has not been reported yet as far as we know [8] , and very few examples of stable Au(III)-diacetylide complexes appear in the literature [37] , [38] . This lack of precedents for Au(III)-diacetylides might indicate that the reactivity of the alkynes once σ-bound to Au(III) is very high, including a potential reductive elimination. It has been proposed that the reductive elimination from a tetracoordinated planar Au(III) complex is favoured respect to other metals [33] since it leaves behind a two-coordinated Au(I) complex stabilized by relativistic effects [39] , [40] , [41] . To study the reductive elimination of alkynes from Au(III) and also if the distal size selectivity occurs at this stage, the Au(III) complex PPh 3 AuCl 3 was prepared [42] and the corresponding Au(III) acetylide complex of 1-dodecyne 1b was forced to be formed [43] . To do that, n -BuLi was added to 1-dodecyne 1b in tetrahydrofurane (THF)- d 8 at −78 °C and the resulting solution was added to PPh 3 AuCl 3 suspended (not soluble) in THF- d 8 at room temperature (2 equiv. of lithium acetylide with respect to gold). The result is shown in Fig. 4a . The bright-yellow complex PPh 3 AuCl 3 became immediately (<1 min) colourless and soluble. 31 P NMR spectroscopy of the solution just after addition of the acetylide solution shows the complete disappearance of the original signal of PPh 3 AuCl 3 (42 p.p.m.) and the appearance of a new single peak at 33 p.p.m. that could correspond to AuPPh 3 Cl. Addition of n -hexane to the THF solution precipitates a white solid that by isolation and characterization with 1 H and 31 P NMR spectroscopy was confirmed to be AuPPh 3 Cl, the corresponding phosphine peak being observed during reaction. Analysis by GC–MS of the n -hexane supernatant shows that the homocoupling C 12 product 2b is the only alkyne product of the reaction, no traces of free 1-dodecyne 1b being present. A similar result is obtained when PPh 3 AuCl 3 is treated with the lithium acetylide of 1-decyne 1a since AuPPh 3 Cl and the C 10 homocoupling product 2a are the only products of the reaction. These results indicate that the reductive elimination of two acetylide fragments from a single Au(III) atom is very fast, in accordance with recent precedents in the literature that reports the efficient formation of C sp 2–C sp 2 bond with Au(III) via reductive elimination at −52 °C reaction temperature [30] . Thus, we must conclude that the distal size selectivity does not occur during the final reductive elimination but occurs in an intermediate step between oxidation and reductive elimination, since reductive elimination of the two alkyne molecules from Au(III) is extremely fast and does not give any distal size selectivity. 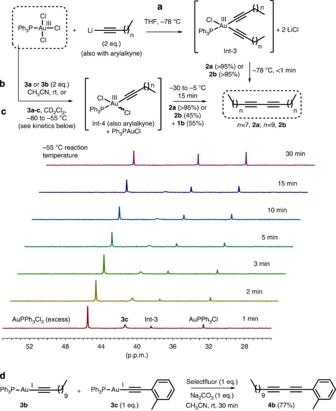Figure 4: Studies on the reductive elimination step. The top schemes (a–c) show the reductive elimination or transmetallation between gold and/or lithium acetylides in stoichiometric amounts. GC yields refer after extraction of the reaction mixture withn-hexane and addition of dodecane as an external standard. The kinetics at low-temperature of the transmetallation of tolylacetylene from3cto an excess (3 equiv.) of AuPPh3Cl3, followed by31P NMR, is also included. Spectra were recorded every 30 s after 1 scan (2.5 s), and a total of 60 measurements were taken. Thein situoxidation and transmetallation of gold(I) alkyl and aryl acetylides is shown at the bottom (d). Figure 4: Studies on the reductive elimination step. The top schemes ( a – c ) show the reductive elimination or transmetallation between gold and/or lithium acetylides in stoichiometric amounts. GC yields refer after extraction of the reaction mixture with n -hexane and addition of dodecane as an external standard. The kinetics at low-temperature of the transmetallation of tolylacetylene from 3c to an excess (3 equiv.) of AuPPh 3 Cl 3 , followed by 31 P NMR, is also included. Spectra were recorded every 30 s after 1 scan (2.5 s), and a total of 60 measurements were taken. The in situ oxidation and transmetallation of gold(I) alkyl and aryl acetylides is shown at the bottom ( d ). Full size image Gold is the most electronegative metal of the periodic table and, consequently, transmetallation of carbon ligands from Au(I)–C and Au(III)–C bonds to other metals is favoured and well-reported in the literature [44] , [45] , [46] . However, transmetallation from Au(I) to Au(III) is scarcely reported [29] although the migration of a carbon ligand from the more electronegative Au(I) to the more electropositive Au(III) cation should be favoured. Figure 4b shows the results obtained when the C 10 Au(I) acetylide 3a was mixed with the Au(III) complex PPh 3 AuCl 3 in acetonitrile. In this case, the homocoupling product 2a is formed as only alkyne product in <5 min at room temperature. This result suggests that the transmetallation of the C 10 acetylide fragment of Au(I) complex 3a to the Au(III) cation readily occurs. When the C 12 Au(I) acetylide 3b was used, the homocoupling product 2b was obtained together with free 1-dodecyne 1b , as described before. To better study this step, we followed the reaction of PPh 3 AuCl 3 with 3a (C 10 ) or 3b (C 12 ), and also with Au(I) arylacetylide 3c (PPh 3 Au- ortho- tolylacetylene), by means of low-temperature 31 P NMR spectroscopy ( Fig. 4c and kinetics). For doing that, the NMR tube containing a solution of PPh 3 AuCl 3 in CD 2 Cl 2 was placed in liquid nitrogen (−196 °C) and then a solution of the corresponding Au(I) acetylide 3a–c in CD 2 Cl 2 , cooled at −78 °C (acetone-dry ice), was slowly added into the NMR tube. After that, the tube was rapidly transferred to the NMR equipment at −80 °C, and measurements were started after shimming. It was found that 3a or 3b react with PPh 3 AuCl 3 in <5 min at −80 °C to give 0.5 equiv. of PPh 3 AuCl and 0.5 equiv. of an unknown phosphine product at 38 p.p.m. and that this intermediate ( Int-4 ) is stable at least up to −30 °C. No differences between 3a (C 10 ) and 3b (C 12 ) were found here. When the NMR tube was left to warm, the only peak found by 31 P NMR was that corresponding to PPh 3 AuCl. 1 H and 13 C NMR confirmed the formation of the homocoupling product 2a from 3a and the mixture of 1b and 2b from 3b . The reaction of PPh 3 AuCl 3 with 3c proceeds slower and a more accurate kinetics could be carried out at −55 °C. Again, PPh 3 AuCl and the unknown peak at 38 p.p.m. were the only products formed in equimolecular amounts. In situ 1 H measurements of the reaction mixture at −55 °C showed a new peak at 2.40 p.p.m. downshifted −0.05 p.p.m. from the original methyl group of the Au(I) tolylacetylide 3c (2.45) and also downshifted (−0.11 p.p.m.) from the homocoupled product (2.51). It is perhaps more informative the result obtained by in situ 13 C NMR measurement at −55 °C. It was found that new peaks corresponding to the arene ring of the alkyne appear and that they present the typical J C – P of the phosphine Au-acetylide complexes and, consistently, that the methyl peak is also shifted with respect to the starting material. The 13 C NMR spectrum strongly suggests that the unknown species at 38 p.p.m. is a new phosphine Au-acetylide that, according to the formation of 1 equiv. of AuPPh 3 Cl per molecule of 3c consumed, it might correspond to PPh 3 Au(III)-tolylacetylene. A similar result is found when lithium tolylacetylide is used. The downshift of the methyl group in 1 H NMR points also in that direction. To further assess if Int-4 is the result of one alkyne transmetallation from 3c to PPh 3 AuCl 3 , the reaction was carried out with an excess (3 equiv.) of the latter to maximize monotransmetallation. Kinetics of the reaction in Fig. 4 gives an initial rate of 0.28 s −1 . In situ 1 H and 13 C measurements of the reaction mixture at −55 °C after consumption of the Au(I) acetylide 3c gave neat spectra with the same phosphine intermediate found above. As for 3a and 3b , this intermediate is stable up to −5 °C and only at this temperature it starts to further convert into PPh 3 AuCl. The kinetic results together with the stoichiometry of the reaction suggest that the gold(I)-acetylides 3a–c transfer the first alkyne group to the Au(III) atom of PPh 3 AuCl 3 at low temperature (−80 °C for alkyl, −55 °C for aryl) to give the intermediate Int-4 PPh 3 Au(III)-alkyne and that the second alkyne transfers at much higher temperature (−30 to −5 °C) to give Int-3 . As soon as Int-3 is formed, reductive elimination occurs and the homocoupling product is released. This means that the transmetallation of the second alkyne is much slower than the transmetallation of the first alkyne, since the former occurs at much higher temperature, and that the reductive elimination is in turn much faster than the second alkyne transmetallation, which correlates well with the results observed with lithium acetylides. In short, these results show that Int-4 is an intermediate of the reaction and that it could very well occur that the mixture of Au(I) acetylide and Int-4 is responsible for the distal size selectivity observed. To mimic better the gold-catalysed system when having separated Au(III) and Au(I) acetylides, and to avoid the use of PPh 3 AuCl 3 , we made use of the different rates of oxidation with selectfluor of alkyl and aryl acetylides. It was shown above that the oxidation of the alkyl acetylide complexes 3a–b (monogold) and 6a–b (digold) by selectfluor proceeds in ~30 min, and we have previously shown that the same oxidation for PPh 3 Au- ortho- tolylacetylene 3c takes place in ~4 h [17] . Thus, in principle, the addition of selectfluor to a mixture of an Au(I) alkyl acetylide and an Au(I) aryl acetylide should oxidize first the alkyl Au(I) complex and form the corresponding Au(III) alkyl acetylide. Once the Au(III) alkyl acetylide is formed, the Au(I) aryl acetylide can transmetalate. It is true that while the oxidation with selectfluor occurs, the remaining Au(I) alkyl acetylide (not oxidized yet) could compete with the Au(I) aryl acetylide to transmetalate. To avoid the self-coupling of the alkyl acetylide, we employed 3b (C 12 ), since the rate of homocoupling is the lowest in the alkyl series and it should not compete with the aryl acetylide. Thus, the Au(I) alkyl acetylide 3b and PPh 3 Au- ortho- tolylacetylene 3c were mixed in the same flask and then selectfluor was added. The result in Fig. 4d shows that the heterocoupled product 4b is the major product of the reaction with a 77% yield, indicating that the transmetallation from Au(I) aryl acetylides to Au(III) alkyl acetylides readily occurs. With the hope that the digold intermediate of unreactive 1-dodecyne could be trapped and characterized, we carried out the oxidation of complex 6b with selectfluor at −78 °C in a CD 2 Cl 2 /CD 3 CN solvent mixture. The results ( Supplementary Fig. 8 ) show the desymmetrization of the original H and P peaks of 6b into two new signals, which points to the formation of the divalent-mixed Au(I,III) complex. Complex 6b was independently prepared without one of the dodecylide fragments and its 31 P NMR signal fits well with the one detected after oxidation of 6b by selectfluor, which supports that one of the dodecylide fragments of 6b leaves as soon as one Au(I) atom is oxidized to Au(III). With all the above results, we can suggest that the distal size selectivity occurs just before the transmetallation step of one alkyl acetylide fragment from Au(I) to Au(III), during the formation of the mixed-valence digold (I,III) complex. The tetracoordinated planar Au(III) site and the linear Au(I) site impose a parallel disposition of the aliphatic chains of each acetylene, which resembles the formation of a highly stabilized self-assembled monolayer, in this case just via two contiguous aliphatic chains. For longer chains, their interaction is enhanced thus blocking the coupling of the alkynes, while for shorter chains the lateral interaction is weak and the reaction readily occurs. 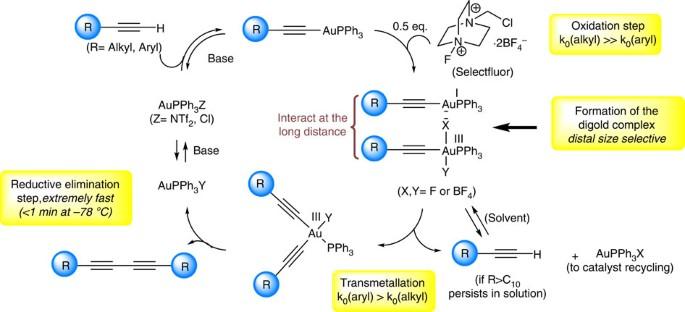Figure 5: Proposed mechanism for the gold-catalysed homocoupling of alkynes with distal size selectivity. The formation of a Au(I)/Au(III) digold intermediate is responsible for the distal steric differentiation. Mechanism of gold-catalysed distal-selective alkyne coupling Figure 5 shows the proposed mechanism to explain the origin of size selectivity during the gold-catalysed homocoupling of alkynes. Figure 5: Proposed mechanism for the gold-catalysed homocoupling of alkynes with distal size selectivity. The formation of a Au(I)/Au(III) digold intermediate is responsible for the distal steric differentiation. Full size image First, the linear Au(I) acetylide complex suffers the oxidation by selectfluor to give the corresponding Au(III) complex. This oxidation is favoured by a second neighbouring Au(I) acetylide molecule in solution but no size selectivity is found for this process, since selectfluor oxidation occurs at a similar rate for both C 10 and C 12 gold acetylides. At this point, we propose an Au(I)/Au(III) intermediate with a congested structure as responsible for the distal size selectivity observed, where the tetracoordinated planar Au(III) acetylide and the dicoordinated linear Au(I) acetylide present a parallel disposition of the aliphatic chains of each acetylene, which resembles the formation of a highly stabilized self-assembled monolayer. This intermediate is supported here experimentally by the similarity of the results obtained with the digold complexes 5a–b and the corresponding acetylides of 5b (complexes 6a–b ), since these complexes have a locked cisoid conformation of acetylides and phosphines. Notice that this particular steric scenario, created by the interaction of a tetracoordinated planar metal complex and a linear metal complex, cannot be found in any metal redox pair of the periodic table but only in Au(I)/Au(III) [40] . In addition, this Au(I)/Au(III) intermediate suitably accommodates acetylides fully substituted in contiguous positions to the triple bond such as tert -butylacetylene 1c , which explains the feasibility of couplings with hindered alkynes around rather than along the triple bond. The experimental results also suggest that protodeauration competes with the transmetallation of the linear alkyl acetylide from Au(I) to Au(III), and that free acetylene is also released after decomposition of the fully oxidized gold acetylide. The alkyne can rebind to the Au(I) atom and enter back into the catalytic cycle provided the acetylide is still active. Gold-catalysed heterocoupling of alkynes The heterocoupling of terminal alkynes has been reported in the literature with different copper catalysts but, in all cases, a five-times amount of one of the alkynes must be added to achieve good yields of heterocoupling product [47] , [48] , [49] , [50] . Otherwise, with a one-to-one molar ratio of alkynes, a statistical 1:2:1 molar ratio of homo:hetero:homocoupled products, or a 1:1:1 molar ratio in some cases, is obtained [47] , [48] , [49] , [50] . In addition, the two alkynes must be differentiated either electronically (aryl or heteropropargyl versus alkyl alkynes, activated versus deactivated aryl alkynes) or sterically near the triple bond (linear versus bulky alkynes). The high excess of one of the alkyne reactants together with the need of electronic and/or steric differentiation of the terminal triple bond limits severely the application of these methodologies in organic synthesis. A much better methodology would consist in a catalytic system able to couple two different terminal alkynes regardless of the nature of the terminal triple bond and without the need of adding an excess of one of them. When we carried out the heterocoupling of different alkynes in equimolecular amounts under the present gold-catalysed conditions, we found that the heterocoupling products were formed in moderate to good yields and with high selectivity ( Supplementary Fig. 9 ) [51] , [52] . One must not be surprised with these results when considering the high yield of heterocoupling obtained when we mix the C 12 Au(I) alkyl acetylide 3b and PPh 3 Au- ortho- tolylacetylene 3c (see Fig. 4d above). If we compare the initial rate of oxidation for the Au(I) alkyl acetylides (220 h −1 , see above) with that of the aryl acetylide (45 h −1 ) [17] , a five-times relationship k 0 (alkyl)/ k 0 (aryl)= k rel (oxidation)≈5 is found. However, the initial reaction rate for the homocoupling of 1-decyne 1a under the gold-catalysed reaction conditions indicated above ( Fig. 1 ) is approximately three times lower than that for ortho -tolylacetylene 1e (ref. 17 ), k 0 (alkyl)/ k 0 (aryl)= k rel (homocoupling)=0.36. Therefore, the rate of oxidation of Au(I)-acetylide and the rate of formation of homocoupling product are decoupled for alkyl and aryl alkynes, with an estimated value of k rel (oxidation)/ k rel (homocoupling)≈14. Since the last step, the reductive elimination from Au(III) is extremely fast (less than a minute at −78 °C) for both alkyl and aryl alkynes, the cross-coupling of aryl and alkyl terminal alkynes is favoured under the present gold-catalysed conditions. Not only that, but the cross-coupling between two different aryl alkynes and also between two different alkyl alkynes is also performed. The coupling of two different alkynes based on gold-catalysed conditions opens a reactivity window for carrying out oxidative heterocouplings of terminal alkynes in 1:1 molar ratio with yield and selectivity clearly beyond the statistical range [53] , [54] . A near atomically precise distal size selectivity occurs during the oxidative coupling of terminal alkynes under gold-catalysed conditions. The formation of a crowded Au(I)/Au(III) digold intermediate is responsible for the distal steric differentiation. Oxidation by selectfluor, transmetallation and reductive elimination do not produce distal size selectivity. The reductive elimination of two alkynes from a single Au(III) atom is extremely fast and occurs in less than a minute at −78 °C. The subtle steric and electronic discrimination of alkynes by this gold-catalysed system allows the heterocoupling of two different alkynes in equimolecular amounts regardless of the nature of the terminal triple bond. How to cite this article: Leyva-Pérez, A. et al. Unique distal size selectivity with a digold catalyst during alkyne homocoupling. Nat. Commun. 6:6703 doi: 10.1038/ncomms7703 (2015).